Constraining timescales of focused magmatic accretion and extension in the Afar crust using lava geochronology As continental rift zones mature the tectonic and volcanic processes associated with crustal extension become confined to narrow magmatic rift zones, reminiscent of oceanic spreading ridges. The formation of these rift zones and the development of ocean-ridge type topography is a significant milestone in rift evolution as it signifies the localization of crustal extension and rift-related volcanism. Here we show that lavas, which erupted since ~200 ka along part of the on-land Red Sea rift system in Afar, Ethiopia, have a consistent age-progression from the rift axis outwards, indicating that axial dyke intrusion has been the primary mechanism of segment growth and that focused magmatic accretion and extension in the crust have remained stable here over this period. Our results suggest that as this rift segment has formed, in thinned and intruded continental crust, the time-averaged surface opening rate has closely approximated the total extension rate between Africa and Arabia. In Afar, Ethiopia, late-stage continental break-up is characterized by the formation of en-echelon magmatic rift zones ( Fig. 1 ), representing focused zones of dyke intrusion, volcanism and faulting [1] . At crustal levels the magmatic and tectonic process operating at these segments closely resemble those observed at slow-spreading ocean ridges [2] , [3] , [4] , [5] and axial dyke intrusions appears to have a key role in accommodating extension [4] and creating characteristic ridge topography [6] . The development of these narrow zones of faulting and magma intrusion signifies an important stage of rift evolution, where extensional processes and volcanic accretion become localised [1] and final stages of crustal thinning may occur before plate rupture and true oceanic spreading [7] . Geodetic studies indicate that in the southern Red Sea all Afro-Arabian extension of 16–20 mm per year is currently accommodated on-land within Afar [8] and the limited magnetic data available suggest that the correlated linear magnetic anomalies, characteristic of oceanic rifts, may have begun forming across the axis of these on-land rift systems, indicating long-term focused volcanic accretion [9] , [10] . 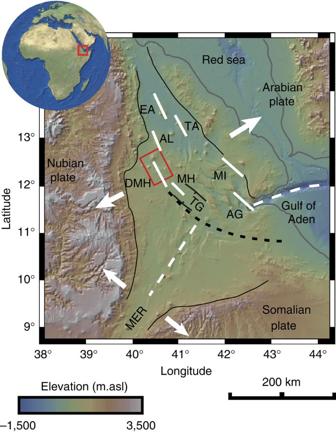Figure 1: Topography and tectonics of Afar. Rifting along the on-land sections of the Red Sea and Gulf of Aden rift systems (north of the Main Ethiopian Rift (MER)), have led to formation of segmented zones of focused faulting and magmatism. EA, Erta Ale; TA, Tat Ali; AL, Alayta; DMH, Dabbahu-Manda Hararo; MH, Manda Hararo; MI, Manda Inakir; AG, Asal-Ghoubbet; TG, Tendaho Graben. Figure 1: Topography and tectonics of Afar. Rifting along the on-land sections of the Red Sea and Gulf of Aden rift systems (north of the Main Ethiopian Rift (MER)), have led to formation of segmented zones of focused faulting and magmatism. EA, Erta Ale; TA, Tat Ali; AL, Alayta; DMH, Dabbahu-Manda Hararo; MH, Manda Hararo; MI, Manda Inakir; AG, Asal-Ghoubbet; TG, Tendaho Graben. Full size image A recent phase of active magmatic rifting (2005–2010) along the Dabbahu-Manda Hararo (DMH) Rift Zone in central Afar (~12.4°N, 40.5°E; Figs 1 and 2 ) has demonstrated the critical importance of axial dyke intrusions in accommodating crustal extension across magmatic segments [3] , [4] . Observations of the multiple (~14) dyke intrusions [3] , [11] , [12] , [13] , [14] , [15] , [16] , [17] and fissure eruptions [18] during this active phase have shown that in the upper part of the crust, the delivery of melts to the DMH rift zone is currently strongly focused along the rift axis. The overall scale and morphology of this ~15 × 60 km magmatic segment is similar to a slow (~20 mm per year) spreading mid-ocean-ridge segment [6] , such as those found along the Mid-Atlantic ridge [19] , [20] , and the recent episodic rifting activity is similar to that previously observed in Iceland [4] , [21] . The formation of the DMH segment is broadly constrained by regional K-Ar geochronological studies to have occurred since ~1 Ma, following a period of widespread fissural volcanism in Afar between ~1–3 Ma (ref. 22 ). Measurements of seismic anisotropy shows a preferred orientation for crustal fabrics that trends parallel to the rift axis, implying that the growth of this rift zone has probably been dominated by axially aligned magma intrusion rather than crustal stretching [23] . 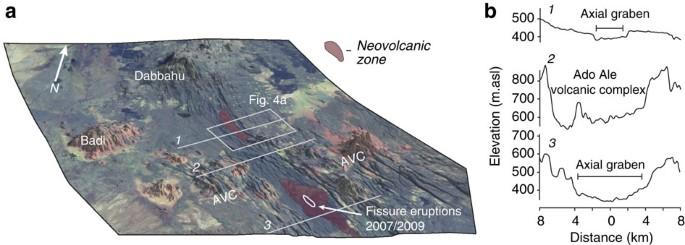Figure 2: Topographic map of the DMH magmatic segment. (a) False colour Landsat ETM+ image of the DMH rift segment. The ~15 × 60 km segment is defined by a zone of closely spaced faulting and recent volcanism. The neovolcanic zone (red area) is recognized from accumulations of recent basaltic lavas (based on flow morphology), which have been concentrated in the axial graben on the northern and southern sides of the Ado Volcanic Complex (AVC). Rhyolitic and trachytic lavas forming parts of the AVC and Badi appear red in colour, basaltic lavas forming the rift floor are dark grey. (b) Across axis topography (lines of sections shown in 2a). Significant variations occur in segment morphology between the southern and northern sectors. Figure 2: Topographic map of the DMH magmatic segment. ( a ) False colour Landsat ETM+ image of the DMH rift segment. The ~15 × 60 km segment is defined by a zone of closely spaced faulting and recent volcanism. The neovolcanic zone (red area) is recognized from accumulations of recent basaltic lavas (based on flow morphology), which have been concentrated in the axial graben on the northern and southern sides of the Ado Volcanic Complex (AVC). Rhyolitic and trachytic lavas forming parts of the AVC and Badi appear red in colour, basaltic lavas forming the rift floor are dark grey. ( b ) Across axis topography (lines of sections shown in 2a). Significant variations occur in segment morphology between the southern and northern sectors. Full size image Recent studies here have largely focused on the active volcanic and tectonic phenomena associated with the recent active rifting phase and the contemporary mechanisms of strain accommodation along this part of the on-land Red Sea rift system are becoming increasingly well understood (see review by ref. 3 ). However, the timescales associated with the structural and magmatic processes involved in segment formation remain largely unconstrained and it is unclear to what extent magmatic accretion has been focused along the rift axis during this period. This is partly due to the remoteness of this region, but also the analytical challenges associated with obtaining geochronological data for the young basaltic lavas that form the segment surface. In this paper, we present new 40 Ar/ 39 Ar plateau ages for basaltic lavas from the eastern rift flank that provide constraints on the timing of volcanic-tectonic processes and history of focused melt intrusion. 40 Ar- 39 Ar geochronology Lava samples for geochemical and geochronological analysis were collected from the eastern flank of the DMH segment north of the Ado Ale Volcanic Complex (AVC) ( Figs 2a and 4a ). Geochronology of low-K basaltic lavas remains analytically challenging, however meaningful age data can be obtained with suitable analytical techniques ( Methods ). 40 Ar- 39 Ar step-heating experiments were performed on groundmass separates of eight lavas from the rift flank; 4 of which produced age-spectra suitable for plateau age determinations, while the remaining samples produced disturbed age-spectra unsuitable for a plateau age interpretation, most likely due to the effects of 39 Ar recoil during sample irradiation [24] . Age data from the successful step-heating experiments is listed in Table 1 and the age-spectra from the step-heating experiments shown in Fig. 3 . These ages range from ~30 to 200 ka and provide information on recent volcano-tectonic processes during the formation of this segment. Figure 4: Age-distribution of lavas across the DMH rift zone. 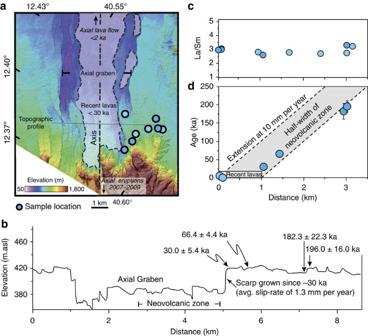Figure 4: Age-distribution of lavas across the DMH rift zone. (a) LiDAR topographic map of part of the DMH magmatic segment showing the location of lava samples. The neovolcanic zone is defined by accumulations of recent lavas (shaded white) in the axial graben, which are constrained by our new age data to be <30 ka. Symbols show locations of samples across rift flank (dark blue symbols are those with new40Ar-39Ar ages). (b)40Ar-39Ar ages from the eastern rift flank projected onto a topographic section. (c) La/Sm versus distance from the rift axis (data from ref.29and S. Medynski, personal communication). (d) Age-distance plot for lavas with40Ar/39Ar ages (>30 ka) and with known ages from the axial graben. The observed age-distribution can be explained by extension from the centre of the current neovolcanic zone (and location of recent dyke intrusions since 2005) at a velocity close to current Afro-Arabian half rate of 10 mm per year. ‘Zero-age’ samples are from axial eruptions in the southern part of the rift between 2007–2009 (ref.18) and from one flow in the northern section with a cosmogenic3He exposure age of <2 ka (S. Medynski, personal communication25). ( a ) LiDAR topographic map of part of the DMH magmatic segment showing the location of lava samples. The neovolcanic zone is defined by accumulations of recent lavas (shaded white) in the axial graben, which are constrained by our new age data to be <30 ka. Symbols show locations of samples across rift flank (dark blue symbols are those with new 40 Ar- 39 Ar ages). ( b ) 40 Ar- 39 Ar ages from the eastern rift flank projected onto a topographic section. ( c ) La/Sm versus distance from the rift axis (data from ref. 29 and S. Medynski, personal communication). ( d ) Age-distance plot for lavas with 40 Ar/ 39 Ar ages (>30 ka) and with known ages from the axial graben. The observed age-distribution can be explained by extension from the centre of the current neovolcanic zone (and location of recent dyke intrusions since 2005) at a velocity close to current Afro-Arabian half rate of 10 mm per year. ‘Zero-age’ samples are from axial eruptions in the southern part of the rift between 2007–2009 (ref. 18 ) and from one flow in the northern section with a cosmogenic 3 He exposure age of <2 ka (S. Medynski, personal communication [25] ). 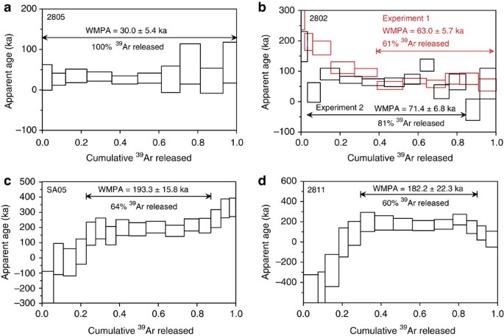Full size image Table 1 40 Ar/ 39 Ar ages for basaltic lavas from the DMH segment. Figure 3:40Ar-39Ar plateau age diagrams. (a–d) Plots show age-spectra obtained from step-heating experiments versus cumulative39Ar gas released. Arrows show heating steps used for plateau age determinations. Data from two separate experiments are shown for sample 2,802. The interpreted age for this sample (listed inTable 1) is a weighted mean of the two plateau ages shown. WMPA stands for weighted mean plateau age. SeeTable 1,MethodsandSupplementary informationfor further details. Full size table Figure 3: 40 Ar- 39 Ar plateau age diagrams. ( a – d ) Plots show age-spectra obtained from step-heating experiments versus cumulative 39 Ar gas released. Arrows show heating steps used for plateau age determinations. Data from two separate experiments are shown for sample 2,802. The interpreted age for this sample (listed in Table 1 ) is a weighted mean of the two plateau ages shown. WMPA stands for weighted mean plateau age. See Table 1 , Methods and Supplementary information for further details. Full size image The DMH segment has a well-defined axial graben offset from the rift flanks by fault scarps 30–100 m high ( Fig. 2b ). Along the rift axis the graben is disrupted by the volcanic topography associated with the Ado Ale Volcanic complex (AVC), a series of faulted silicic lavas flows/domes on the rift flanks and a basaltic volcano at the rift axis with a summit crater, and at its northern end the Dabbahu volcano, which has been active since at least ~80 ka (refs 25 and (S. Medynski personal communication) [25] , [26] ). Seismic [11] , [12] , [13] and geodetic [14] , [15] , [16] , [17] observations of the recent dyking events are consistent with a magma source located in the rift centre below the AVC. This central volcanic region also marks a division in the width and morphology of the axial graben and rift flanks between the southern (graben ~8 km wide, scarps ~100 m high, significant flank topography) and northern (graben ~4 km wide, scarps ~30–50 m high, smooth flank profile) sectors ( Fig. 2b ). Morphological evidence shows that the most recent volcanism has been contained within the axial graben, concentrated on the northern and southern sides of the central basaltic edifice (region coloured red in Fig. 2a ). These lavas define a 2–3 km wide neovolcanic zone across the graben centre, which is similar in scale to that found along parts of the mid-Atlantic ridge [26] . Structural evidence from faulting observed during the recent active period suggests that at the rift surface brittle deformation is largely controlled by dyke intrusion and close links, therefore, exists between magmatism and segment morphology [6] . One of the flows in our new geochronological data set is offset by the main graben bounding fault scarp (sample 2,805 30.0±5.4 ka) and constrains the growth of this ~40 m high fault scarp to <30 ka, with a time-averaged slip rate of ~1.3 mm per year ( Fig. 4b ). In the northern sector, the growth of this scarp is linked to the formation of the current axial graben, which is shown to be relatively young. Unlike in the southern sector (that is, south of the AVC) large fault scarps are not evident across the northern rift flanks and large-offset faults have either not previously formed here or these have been covered by volcanic infilling. Our new age data provides a maximum age for the present day eastern scarp, however it remains unclear if the growth of this scarp since ~30 ka is the result of increased slip-rates or a decrease in volcanic re-surfacing. As recent volcanism has been essentially confined to the axial graben (based on flow morphology, axial eruptions since 2007 (ref. 16 )) and one 3 He exposure age of <2 ka (S. Medynski, personal communication; Figs 2a and 4a ) our new age data implies that these flows forming the present the neovolcanic zone have a maximum age of ~30 ka. The oldest lavas in our geochronological data set were sampled ~2 km from the edge of the graben and have 40 Ar- 39 Ar plateau ages of 196.0±16.0 ka and 182.3±22.3 ka. A sample between these and the youngest dated flow gives an intermediate age of 66.4±4.4 ka (weighted mean of plateau ages from two heating experiments; Fig. 3 and Table 1 ). Although deformation of these flows by normal faulting currently prevents the reconstruction of individual eruptive systems, and it is, therefore, not possible to precisely locate the paleo-eruptive fissures, potential flow lengths can be estimated from the width of the current neovolcanic zone (assuming axial emplacement). Using this width as proxy for the uncertainty of the paleo-emplacement zone, the observed age-distribution of all lavas with known ages across the rift segment shows a good correlation to a model of emplacement in the axial graben and subsequent transport outwards at a velocity of ~10 mm per year ( Fig. 3d ), close to the predicted long-term Afro-Arabian half-rate [8] , [27] . These results suggest that since ~200 ka volcanism in the main rift zone has been primarily focused along the axial graben, demonstrating long-term focused magmatic accretion. The long-term extension rate implied by our age-profile is consistent with the recent rifting activity observed here, which suggests that crustal deformation and extension along the incipient African-Arabian plate boundary occurs via discrete magmatic episodes, focused along the segment axis [3] , [4] . This model of segment growth is supported by geochemical data for these lavas (ref. 28 and S. Medynski, personal communication), which shows that lavas sampled from the axis outwards (shown in Fig. 4a ) have a limited compositional range ( Fig. 4c ) and are distinct from those erupted at other nearby volcanoes (that is, the Dabbahu volcano and volcanic vents west of the main segment; Fig. 2 ). Recent dyke intrusions have been principally fed by melts sourced from the mid-segment magma reservoir beneath the AVC and the compositional similarity between the recent fissural basalts and lavas sampled across the rift flanks (as shown in Figs 4c and 5 ) suggests that this centralized supply has been feeding axial intrusions over the last ~200 ka of segment growth. 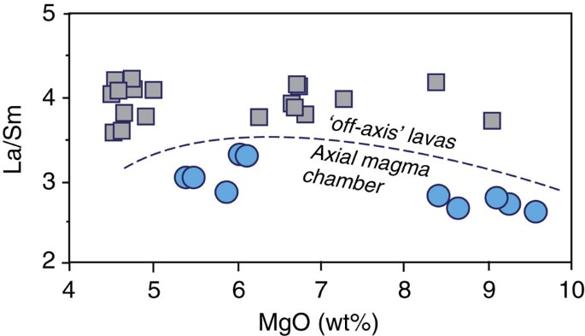Figure 5: La/Sm versus MgO for lavas from the DMH segment and nearby volcanoes. A clear compositional division exists between the lavas that form the main part of the segment (including recently erupted lavas) (blue symbols) and those from other nearby vents and volcanoes (grey symbols; that is, Badi and Dabbahu volcanoes;Fig. 2). Data from ref 28 and S. Medynski personal communication28. Figure 5: La/Sm versus MgO for lavas from the DMH segment and nearby volcanoes. A clear compositional division exists between the lavas that form the main part of the segment (including recently erupted lavas) (blue symbols) and those from other nearby vents and volcanoes (grey symbols; that is, Badi and Dabbahu volcanoes; Fig. 2 ). Data from ref 28 and S. Medynski personal communication [28] . Full size image The new age data presented here for lavas from the DMH rift zone indicate a systematic age-distance trend from the rift axis, consistent with a model of segment formation via focused axial dyke intrusion and volcanic accretion since at least ~200 ka. The observed age-distribution across the rift flanks implies that during this period the long-term time-averaged opening rate at this rift zone has closely approximated the total estimated extension rate between Africa and Arabia and strain accommodation has, therefore, been focused here over this period. The composition of the lavas that form the surface of the main part of the segment is consistent with a common source to the recent fissural basalts [18] , and supports the existence of a long-lived centralized melt supply. Focused magmatic accretion in the crust can, therefore, remain stable over a kilo-year timescale before marked crustal thinning. Future work involving detailed structural investigations and further geochronological analysis will build upon the constraints presented to develop understanding of how this and other mature rift systems develop during the latter phases of continental break-up. 40 Ar- 39 Ar geochronology Samples were first inspected in thin section to select those with textures that were as close to holocrystalline and equigranular as possible and to identify the appropriate size fraction required for a groundmass separate. Selected samples were then crushed and sieved to collect the desired size fraction. This was then thoroughly cleaned in an ultrasonic bath with successive rinses of DI water and isopropyl alcohol. After cleaning samples were passed through a FRANTZ magnetic separator to increase the proportion of groundmass to phenocryts. Around 250 mg of groundmass material was then handpicked using a binocular microscope. For irradiation, ~250 mg groundmass sample were packaged in Cu foil and placed in a cylindrical quartz vial, together with fluence monitors of known age and K-glass, and fluorite to measure interfering isotopes from K and Ca. The quartz vials were wrapped in 0.5 mm-thick Cd foil to shield samples from thermal neutrons during irradiation. The samples were irradiated for one (IRR279) or two (IRR276) hours in the central thimble of the US Geological Survey TRIGA reactor in Denver, Colorado [29] . The reactor vessel was rotated continuously during irradiation to avoid lateral neutron flux gradients. Reactor constants determined for these irradiations were indistinguishable from recent irradiations, and a weighted mean of constants obtained over the past 5 years yields 40 Ar/ 39 Ar K =0.0010±0.0004, 39 Ar/ 37 Ar Ca =0.00071±0.00005, and 36 Ar/ 37 Ar Ca =0.000281±0.000006. TCR-2 sanidine from the Taylor Creek Rhyolite [30] was used as a fluence monitor with an age of 27.87 Ma. This monitor is a secondary standard calibrated against the primary intra-laboratory standard, SB-3, that has an age of 162.9±0.9 Ma (ref. 31 ). Fluence monitors were analysed using a continuous CO2 laser system and mass spectrometer described by [32] . Argon was extracted from groundmass and mica separates using a Mo crucible in a custom resistance furnace modified from the design of [33] attached to the above mass spectrometer. Heating temperatures were monitored with an optical fibre thermometer and controlled with an Accufiber Model 10 controller. Gas was purified continuously during extraction using two SAES ST-172 getters operated at 4A and 0A. Mass spectrometer discrimination and system blanks are important factors in the precision and accuracy of 40 Ar/ 39 Ar age determinations of Pleistocene lavas because of low-radiogenic yields. Discrimination is monitored by analysing splits of atmospheric Ar from a reservoir attached to the extraction line and for these samples D1amu=1.007504±0.000279. All isotopic ratios are mass discrimination corrected using 40 Ar/ 36 Ar=295.5 (ref. 34 ). A recent determination of atmospheric argon ( 40 Ar/ 36 Ar=298.56±0.31; ref. 35 ) is more precise, but acceptance is controversial and that ratio has no impact on this study because normalizing to a different value does not change the age [36] . Typical system blanks including mass spectrometer backgrounds were 1.5 × 10 −18 mol of m / z 36, 9 × 10 −17 mol of m / z 37, 3 × 10 −18 mol of m / z 39 and 1.5 × 10 −16 mol of m / z 40, where m / z is mass/charge ratio. In the incremental-heating experiments, the extraction line is isolated from pumping systems and the sample is heated to a specified temperature for 10 min, cooled for 3–5 min and transferred to an isolated mass spectrometer. The gas is exposed to getters during the entire extraction. Isotopic ratios are measured and corrected for instrumental blanks, mass discrimination and interfering isotopes generated in the reactor. In these experiments, we separated and loaded enough material to do 12–18 steps on each unknown in order to carefully characterize the argon release. The incremental-heating data are plotted both as an age spectrum diagram and as an isotope correlation (isochron) diagram. For the age spectrum, apparent ages are calculated assuming that non-radiogenic Ar is atmospheric ( 40 Ar/ 36 Ar=295.5) in composition and are plotted against the cumulative 39 Ar released during the experiment. In cases with several contiguous steps yielding ages within analytical error, we calculate and report plateau ages by weighing individual ages by the inverse of their analytical error. Most groundmass age experiments do not yield identical ages across the entire spectrum due to minor alteration, recoil of 39 Ar during irradiation or modest excess 40 Ar. Generally accepted criteria for a meaningful incremental-heating age are; 1: well-defined plateau (horizontal age spectrum) for >50% of the 39 Ar released; 2: well-defined isochron for the plateau gas fractions; 3: concordant plateau and isochron ages; and 4: 40 Ar/ 36 Ar isochron intercept not significantly different from 295.5 (refs 37 , 38 , 39 ). For isochron plots, data are not corrected using an atmospheric ratio. Isochron ages include plateau steps on well-behaved samples or a subset of data that yield a reasonable goodness of fit. We show normal isochron plots for these low-radiogenic rocks because the data are easier to visualize. Inverse isochron results are indistinguishable. Isochron ratios are particularly vulnerable to mobilization of argon isotopes during irradiation [24] , particularly in fine-grained volcanic rocks. 39 Ar produced from 39 K in the reactor recoils ~0.1 μm causing different degassing rates during analysis [24] . Recoil moves ratios along the x -axis of isotope correlation plots with low-T steps moved to lower values (loss of 39 Ar) and high-T steps moved toward higher values (deeply implanted 39 Ar). In this case, the isochron line becomes shallow, yielding a high 40 Ar/ 36 Ar ratio and young isochron age. We interpret this as an irradiation artifact. The most reliable results generally include gas from the middle of the release spectrum with consistent K/Ca ratios and concordant isochron data with 40 Ar/ 36 Ar intercepts within error of air. Reported uncertainties on ages and isotopic ratios are 1σ. Final ages are recalculated to a 28.02 Ma Fish Canyon sanidine age reflecting first principles calibration of GA1550 biotite at 98.8±1.0 Ma (refs 39 , 40 , 41 ). How to cite this article: Ferguson, D. J. et al . Constraining timescales of focused magmatic accretion and extension in the Afar crust using lava geochronology. Nat. Commun. 4:1416 doi: 10.1038/ncomms2410 (2013).